Molecular determinants of common gating of a ClC chloride channel Uniquely, the ClC family harbours dissipative channels and anion/H + transporters that share unprecedented functional characteristics. ClC-1 channels are homodimers in which each monomer supports an identical pore carrying three anion-binding sites. Transient occupancy of the extracellular binding site by a conserved glutamate residue, E232, independently gates each pore. A common gate, the molecular basis of which is unknown, closes both pores simultaneously. Mutations affecting common gating underlie myotonia congenita in humans. Here we show that the common gate likely occludes the channel pore via interaction of E232 with a highly conserved tyrosine, Y578, at the central anion-binding site. We also identify structural linkages important for coordination of common gating between subunits and modulation by intracellular molecules. Our data reveal important molecular determinants of common gating of ClC channels and suggest that the molecular mechanism is an evolutionary vestige of coupled anion/H + transport. ClC proteins serve important physiological functions by mediating the movement of inorganic anions across biological membranes [1] . Surprisingly the ClC family, originally envisaged as entirely composed of electro-diffusive channels, also harbours stoichiometrically coupled anion/H + exchangers [2] , [3] , [4] , [5] , [6] , [7] . Perhaps even more surprisingly, the predictive usefulness of the crystal structure of a prokaryotic ClC Cl − /H + antiporter, ClC-ec1, as a model for ClC channel structure and function shows that these subclasses of ClC proteins share the same basic design [8] , [9] , [10] , [11] . Crystal structures of Cl − /H + antiporters have revealed three distinct anion-binding sites; S ext , S cen and S int (labelled by proximity to the extracellular ( S ext ) and intracellular ( S int ) solutions, respectively), which form the anion transport pathway. The Cl − permeation pathway is capped at the extracellular entrance by a conserved glutamate residue, E ext , and on the intracellular side by a conserved tyrosine residue, Y cen [8] , [12] . Recently Feng et al. [13] have proposed a working model for coupled Cl − /H + transport where the side chain of E ext cycles between S cen , S ext and the extracellular solution. In residence of S cen E ext interacts closely with Y cen and accepts an H + delivered from the intracellular H + transport pathway, and the newly protonated E ext changes conformation to the extracellular solution. In this state S ext and S cen are occupied by Cl − ions from the extracellular solution. Reversion of deprotonated E ext into S cen coincides with transport of these Cl − ions to the intracellular solution, neatly accounting for the 2:1 stoichiometry of Cl − /H + transport. Crucially, a fundamental assumption of this model is that the energetic barriers for Cl − entry and exit from the extracellular side are lower than for the intracellular side. If this were not the case then when E ext does not occupy the pore uncoupled Cl − movement would be possible and the protein would take on the characteristics of a gated Cl − channel [13] . ClC channels are homodimers in which each subunit supports a separate, identical ion-conducting pore [14] , [15] , [16] . The best-characterized ClC proteins are the ‘muscle-type’ channels: ClC-0 and ClC-1. Two gating processes regulate channel activity: separate gates acting on each protopore independently, and a common gate that simultaneously regulates both pores [17] , [18] . ClC-0 common gating occurs over a time course of seconds, ranging to minutes [18] , whereas ClC-1 common gating transitions occur more rapidly [17] . For this reason ClC-0 protopore gating is historically referred to as ‘fast’ gating and common gating as ‘slow’ gating. The structural basis of protopore gating, inferred from prokaryotic Cl − /H + exchanger crystal structures [8] , involves an external gate formed by E ext that opens when protonated [19] to reveal S ext [8] . More widespread conformational changes may accompany protopore gating [20] ; however, their nature is unclear. In contrast the molecular mechanism of common gating is presently obscure. Common gating of ClC-1 channels is medically important because the vast proportion of ClC-1 mutations that cause myotonia congenita affect the voltage dependence of the common gate [21] . Common gating involves widespread [22] , [23] cooperative conformational rearrangements that appear to be communicated across the intersubunit interface [24] . Several lines of evidence suggest that, in addition to its obligate role in protopore gating, E ext is also a critical determinant of common gating. First, common gating of ClC-0 [25] , [26] and ClC-1 [17] depends on Cl − concentration, hinting at the involvement of residues in the channel pore. Second, neutralization of E ext in ClC channels removes both protopore and common gating, resulting in a constitutively open phenotype [8] , [19] , [20] , [27] , [28] , [29] , whereas, in ClC-1 at least, the wider conformational rearrangements consistent with common gating appear to remain intact [23] . Third, mutation of ClC-0 E ext to aspartate (E166D), which mainly differs from glutamate by having a shorter side chain, greatly reduces open probability of the protopore gate while simultaneously locking the common gate open [19] . Fourth, and finally, common gating of ClC-0 E166A and E166D mutant channels could be partially recovered by tandem expression with a WT (wild type) subunit [19] . Remarkably, ClC-0 channels appear to behave as ‘broken’ antiporters, where common gating transitions are linked to H + transport [30] . ClC-0 gating deviates from equilibrium in that closure of the common gate is typically preceded by closure of one of the protopore gates, and the common gate opens to a state where both protopore gates are open [31] . The energy source driving non-equilibrium gating appears to be transport of H + by the common gating mechanism [30] . ClC-1 channels have also been shown to transport H + [6] . In the same experiments Picollo and Pusch [6] did not observe H + transport by ClC-0 channels, which contained a mutation (C212S) that removes common gating [32] . It therefore seems possible that common gating of ClC channels is an evolutionary vestige of the conformational changes that catalyse coupled anion/H + transport [30] . We hypothesized that the model of Cl − /H + transport proposed by Feng et al. [13] may reflect the molecular mechanism of common gating of ClC channels. Our experiments show that, similar to its role as the intracellular gate of ClC-ec1 antiporters [33] , Y cen is an important determinant of ClC-1 and ClC-0 common gating, and is critical for the inhibition of ClC-1 common gating by extracellular Zn 2+ . We also identify a bifurcated salt bridge linking common gating transitions to the subunit interface. In addition we show that Y578 is critical for the modulation of ClC-1 common gating by intracellular NAD + and identify a molecular pathway linking NAD + binding to intracellular CBS domains with conformational changes affecting Y578. Mutations of Y578 affect ClC-1 common gating Molecular modelling, based on the crystallographic coordinates of CmClC, predicted that the phenolic hydroxyl group of Y cen (Y578) directly coordinates Cl − at the central binding site in ClC-1 channels ( Fig. 1 ). Y cen mutations have little effect on Cl − selectivity or conductance of ClC-0 and ClC-1 channels, suggesting a minor role in ion-conduction [10] , [34] , [35] . Instead we hypothesized that Y578 may be an important determinant of ClC-1 common gating. For this reason we refer to our CmClC based model ( Fig. 1c ) as the ‘inactivated’ model in the following text. One observation offered tentative support for our hypothesis. In prokaryotic ClC anion/H + exchange proteins a glutamate residue, corresponding to E203 in ClC-ec1, forms an essential part of the H + transport pathway [36] . This residue is present on helix H, which forms the pseudo-symmetrical dimer interface ( Supplementary Fig. S1 ). Residue E203 is not conserved in ClC-1 ( Supplementary Fig. S1 ); however, mutation of the corresponding valine (V292L) greatly reduces ClC-1 common gating [27] . Comparison of our homology models suggested that interaction with the side chain of V292 might force Y578 to occupy S cen where it would be available to hydrogen bond with E232 ( Fig. 1c ). 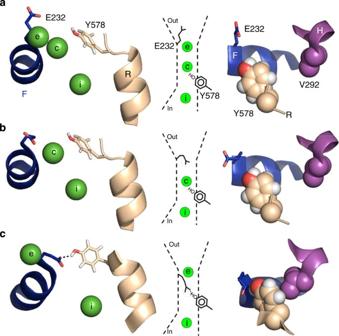Figure 1: Homology models illustrate a possible molecular mechanism for ClC-1 common gating. Shown are ClC-1 models based on homology to the crystallographic coordinates of (a). ClC-ec1 E148Q (PDB id: 1OTU), (b) ClC-ec1 (PDB id: 1OTS) and (c) CmClC coordinates (PDB id: 3ORG). Panels (a) and (b) depict the open and closed conformation of the protopore gate, respectively. Panel (c) depicts the conformation of E232 that we hypothesize corresponds to the closed common gate. Each panel shows: at left, a representation of the pertinent model; middle, a cartoon representation of the relationship between key side chains and anion-binding sites; right, an alternative view depicting the relationship between residues V292 and Y578 for the respective model. Coloured figures show relevant ClC-1 helices as ribbons coloured blue (helix F), yellow (helix R) and magenta (helix I). The side chains of residues E232 (Eext), Y578 (Ycen) and V292 are depicted as sticks, and coloured by atom. Spheres coloured in green depict anion-binding sites,Sext(e),Scen(c) andSint(i), modelled based on respective crystallographic coordinates for each panel. Dashed lines in (c) represent a possible hydrogen bond between the carboxylate group of E232 and the phenolic-hydroxyl group of Y578. For sequence alignments and a structural overview of the protein regions examined in this study please refer toSupplementary Fig. S1. Figure 1: Homology models illustrate a possible molecular mechanism for ClC-1 common gating. Shown are ClC-1 models based on homology to the crystallographic coordinates of ( a ). ClC-ec1 E148Q (PDB id: 1OTU), ( b ) ClC-ec1 (PDB id: 1OTS) and ( c ) CmClC coordinates (PDB id: 3ORG). Panels ( a ) and ( b ) depict the open and closed conformation of the protopore gate, respectively. Panel ( c ) depicts the conformation of E232 that we hypothesize corresponds to the closed common gate. Each panel shows: at left, a representation of the pertinent model; middle, a cartoon representation of the relationship between key side chains and anion-binding sites; right, an alternative view depicting the relationship between residues V292 and Y578 for the respective model. Coloured figures show relevant ClC-1 helices as ribbons coloured blue (helix F), yellow (helix R) and magenta (helix I). The side chains of residues E232 (E ext ), Y578 (Y cen ) and V292 are depicted as sticks, and coloured by atom. Spheres coloured in green depict anion-binding sites, S ext (e), S cen (c) and S int (i), modelled based on respective crystallographic coordinates for each panel. Dashed lines in ( c ) represent a possible hydrogen bond between the carboxylate group of E232 and the phenolic-hydroxyl group of Y578. For sequence alignments and a structural overview of the protein regions examined in this study please refer to Supplementary Fig. S1 . Full size image We tested a panel of Y578 mutant channels to examine the role of this residue in ClC-1 gating. To dissect open probabilities of the protopore ( P o protopore ) and common ( P o common ) gates we used the method determined by Accardi and Pusch [17] , which exploits the different kinetics of the gating processes at very positive voltages ( Fig. 2 ). Protopore gating of Y578A, Y578F, Y578H and Y578K mutants was marginally affected, with the exception of a substantial increase in the minimum value of P o protopore ( V ) for Y578F mutant channels ( Fig. 2b and Supplementary Table S1 ). In contrast the mutations affected ClC-1 common gating by increasing the minimum value of P o common ( V ) and decreasing the apparent gating charge ( Fig. 2c and Supplementary Table S1 ). Mutation Y578E had severe effects on ClC-1 gating and we were unable to fit equation (1) to tail currents recorded from this mutant; as such, data for this mutant are not included in Fig. 2b,c or Supplementary Table S1 . Our results were reminiscent of the effect of Y cen mutations in ClC-ec1, where ability of mutations to uncouple H + transport correlated with the effect on occupancy of S cen [37] . Specifically, Y578A, Y578H and Y578E mutations had the most prominent effects on ClC-1 common gating ( Fig. 2c and Supplementary Table S1 ), just as the corresponding mutations in ClC-ec1 led to strong uncoupling of Cl − /H + transport and reduced anion occupancy of S cen . 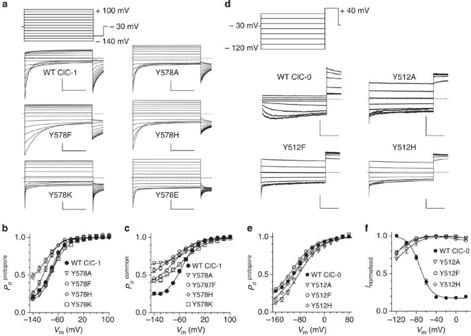Figure 2: Mutations of Ycenaffect ClC-1 and ClC-0 common gating. (a) Voltage protocol for recording ClC-1 channel activity and representative whole-cell current traces for WT ClC-1 and mutants. Dashed lines represent zero-current level and scale bars are 2 nA (vertical) and 100 ms (horizontal). (b) Protopore and (c) common gating curves for WT ClC-1 and Y578 mutants. Open probability of protopore and common gates was dissected using the method described by Accardi and Pusch17. Briefly, apparent open probability (Pochannel) was determined from the tail current amplitude, measured at −100 mV, following application of test voltages (shown in (a)). As the time course of protopore and common gating relaxations are separated by approximately two orders of magnitude at positive voltages it is possible to fully activate the protopore gates, without significantly affecting the common gate, by inserting a brief voltage pulse to +170 mV preceding the tail voltage17. Tail currents recorded using this protocol therefore reflect the open probability of the common gate (Pocommon). Open probability of the protopore gate (Poprotopore) was calculated byPoprotopore=Pochannel/Pocommon. Data points are means±s.e.m. Solid lines represent the fit of equation (1) to the experimental data points.n=4 (WT ClC-1 and Y578K),n=5 (Y578A and Y578F) orn=7 (Y578H). Please refer toSupplementary Table S1for parameters of fits of equation (1). (d) Voltage protocol used to examine ClC-0 common gating and representative whole-cell current traces for WT ClC-0 and mutants. Dashed lines represent zero-current level, and scale bars are 1 nA (vertical) and 1 s (horizontal). (e) Protopore gating of ClC-0 and mutants, calculated from tail current amplitudes, at −100 mV, following a 100 ms test pulse. (f) Common gating of ClC-0 and mutants. Data are current amplitudes at the end of the 0.8 s tail voltage, as shown in (d), normalized to peak current amplitude. Data for (e) and (f) are means±s.e.m. fromn=3 (WT ClC-0), 3 (Y512A), 4 (Y512F) and 4 (Y512H) separate experiments. Figure 2: Mutations of Y cen affect ClC-1 and ClC-0 common gating. ( a ) Voltage protocol for recording ClC-1 channel activity and representative whole-cell current traces for WT ClC-1 and mutants. Dashed lines represent zero-current level and scale bars are 2 nA (vertical) and 100 ms (horizontal). ( b ) Protopore and ( c ) common gating curves for WT ClC-1 and Y578 mutants. Open probability of protopore and common gates was dissected using the method described by Accardi and Pusch [17] . Briefly, apparent open probability ( P o channel ) was determined from the tail current amplitude, measured at −100 mV, following application of test voltages (shown in ( a )). As the time course of protopore and common gating relaxations are separated by approximately two orders of magnitude at positive voltages it is possible to fully activate the protopore gates, without significantly affecting the common gate, by inserting a brief voltage pulse to +170 mV preceding the tail voltage [17] . Tail currents recorded using this protocol therefore reflect the open probability of the common gate ( P o common ). Open probability of the protopore gate ( P o protopore ) was calculated by P o protopore = P o channel / P o common . Data points are means±s.e.m. Solid lines represent the fit of equation (1) to the experimental data points. n =4 (WT ClC-1 and Y578K), n =5 (Y578A and Y578F) or n =7 (Y578H). Please refer to Supplementary Table S1 for parameters of fits of equation (1). ( d ) Voltage protocol used to examine ClC-0 common gating and representative whole-cell current traces for WT ClC-0 and mutants. Dashed lines represent zero-current level, and scale bars are 1 nA (vertical) and 1 s (horizontal). ( e ) Protopore gating of ClC-0 and mutants, calculated from tail current amplitudes, at −100 mV, following a 100 ms test pulse. ( f ) Common gating of ClC-0 and mutants. Data are current amplitudes at the end of the 0.8 s tail voltage, as shown in ( d ), normalized to peak current amplitude. Data for ( e ) and ( f ) are means±s.e.m. from n =3 (WT ClC-0), 3 (Y512A), 4 (Y512F) and 4 (Y512H) separate experiments. Full size image Owing to opposite voltage dependence and vastly different kinetics, protopore and common gating can be more readily dissected in ClC-0. ClC-0 common gating can be monitored in whole-cell records by increased current amplitude at a tail voltage after prolonged hyperpolarization of test voltages ( Fig. 2d ). We therefore examined the effects of Y cen (Y512) mutations on ClC-0 common gating. Mutations Y512F, Y512A and Y512H had little effect on ClC-0 protopore gating ( Fig. 2e ); however, none of the mutants showed hyperpolarisation-activated channel gating ( Fig. 2f ). Tail currents measured at positive voltages suggested that channel open probability decreased after long hyperpolarizing pulses ( Fig. 2f ). However, due to the extremely long voltage pulses in these experiments, and their effect on the distribution of chloride ion, we are unable to draw any firm conclusions from this curious observation. In contrast to the equivalent ClC-1 mutations, both ClC-0 Y512K and Y512E mutants were non-functional, suggesting defective trafficking or protein folding. Our results confirm that Y cen is an important determinant of common gating of ClC channels. Zn 2+ inhibition of ClC-1 Y578 mutants Extracellular Zn 2+ inhibits ClC-0 and ClC-1 channels by binding to and stabilising a closed state of the common gating mechanism [38] , [39] . Previous studies suggest that the binding site for Zn 2+ is at the extracellular surface of helix G, where it intersects helix F in the region of E232 [32] , [39] . Mutations C277S and C278S, at the carboxy-terminal of helix G, greatly reduce Zn 2+ inhibition of ClC-1 (ref. 39 ). Mutations of residue C277 have drastic effects on common gating [40] , [41] . However, the role of C277 in Zn 2+ binding is complicated by the fact that common gating is essentially eliminated in C277S mutant channels [39] , [40] , and therefore reduced Zn 2+ inhibition may reflect the absence of common gating rather than diminished Zn 2+ binding. The role of residue C278 in Zn 2+ binding is more clearly defined, as mutation C278S has little effect on ClC-1 common gating, but essentially abrogates Zn 2+ inhibition [39] . Our modelling studies suggested that the slow time course of ClC-1 inhibition by Zn 2+ may arise due to ‘masking’ of Zn 2+ binding residues on helix G, largely by way of residue F235 on helix F ( Fig. 3a ). In support of this argument removal of the aromatic moiety of F235 had little effect on ClC-1 common gating ( Supplementary Fig. S2 ) but greatly accelerated inhibition of F235L mutant channels by 1 mM extracellular Zn 2+ ( Fig. 3b ). We hypothesized that Zn 2+ traps the conformation where the carboxylate group of E232 is hydrogen-bonded to the phenolic hydroxyl group of Y578, and therefore the time course of Zn 2+ inhibition of Y578 mutants should reflect the favourability of interactions between E232 and the various substituted side chains at residue 578. 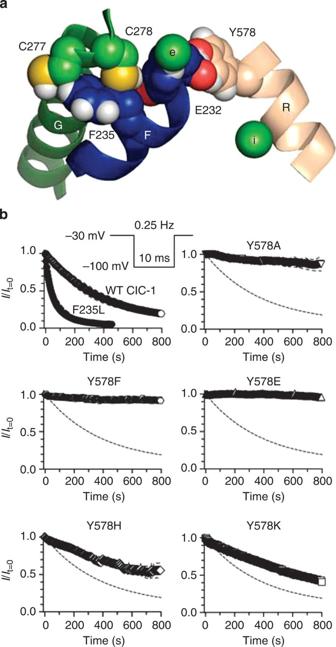Figure 3: Y578 mutations affect Zn2+inhibition of common gating. (a) Relationship between Zn2+-binding residues C277 and C278, residue F235, and residues E232 (Eext) and Y578 (Ycen) in the inactivated ClC-1 homology model, based on EcClC coordinates. In these panels helix G is coloured green and other helices and residues are coloured as inFig. 1(helix F, blue; helix R, yellow). Similarly, anion-binding sites are depicted as green spheres, and are labelledSext(e) andSint(i). (b) Inhibition of WT ClC-1, F235L and Y578 mutant channels by 1 mM extracellular Zn2+. Data points represent peak current amplitude elicited by a 10 ms pulse to −100 mV, applied from a holding potential of −30 mV at 4-s intervals (inset), normalized to current amplitude preceding application of Zn2+. Data are means from WTn=5, F235Ln=4, Y578An=3, Y578Fn=4–5, Y578En=3, Y578Hn=4–12 and Y578Kn=3 (separate experiments). Dotted lines represent s.e.m. Dashed lines representing the fit of a single exponential function with an added minimum asymptote to WT ClC-1 data (τ=378±17 s, minimum asymptote=0.08±0.02) are included in each panel for the purpose of comparison. Representative current traces and gating curves for mutant F235L are shown inSupplementary Fig. S2. Figure 3: Y578 mutations affect Zn 2+ inhibition of common gating. ( a ) Relationship between Zn 2+ -binding residues C277 and C278, residue F235, and residues E232 (E ext ) and Y578 (Y cen ) in the inactivated ClC-1 homology model, based on EcClC coordinates. In these panels helix G is coloured green and other helices and residues are coloured as in Fig. 1 (helix F, blue; helix R, yellow). Similarly, anion-binding sites are depicted as green spheres, and are labelled S ext (e) and S int (i). ( b ) Inhibition of WT ClC-1, F235L and Y578 mutant channels by 1 mM extracellular Zn 2+ . Data points represent peak current amplitude elicited by a 10 ms pulse to −100 mV, applied from a holding potential of −30 mV at 4-s intervals (inset), normalized to current amplitude preceding application of Zn 2+ . Data are means from WT n =5, F235L n =4, Y578A n =3, Y578F n =4–5, Y578E n =3, Y578H n =4–12 and Y578K n =3 (separate experiments). Dotted lines represent s.e.m. Dashed lines representing the fit of a single exponential function with an added minimum asymptote to WT ClC-1 data ( τ =378±17 s, minimum asymptote=0.08±0.02) are included in each panel for the purpose of comparison. Representative current traces and gating curves for mutant F235L are shown in Supplementary Fig. S2 . Full size image Examination of the Zn 2+ sensitivity of Y578 mutants bore out this hypothesis ( Fig. 3b ). In general, Y578 mutants negating a favourable electrostatic interaction with E232; Y578A, Y578F and Y578E were essentially insensitive to extracellular Zn 2+ . Alternatively, positively or partially charged mutants that could interact favourably with E232, Y578K and Y578H were inhibited by Zn 2+ . We also examined mutations of the residue adjacent to Y578, D579, which is not predicted to participate in formation of S cen ( Supplementary Fig. S3 ). In contrast to Y578 mutants, D579N and D579K mutations reduced open probability of the common gate in the voltage range tested, and were robustly inhibited by Zn 2+ ( Supplementary Fig. S3 ). A bifurcated salt bridge is important for ClC-1 gating Coordination of ClC-1 common gating between subunits occurs across the subunit interface, in no small part by intersubunit interactions between helices H and I [24] , [27] . Our results suggested that closure of the common gate coincides with a conformational rearrangement at the extracellular junction of helices G and F, creating a Zn 2+ -binding site, and simultaneously promoting a conformation of E232 where it is able to hydrogen bond with Y578. Helix G forms contacts with helix F (carrying E232 at its amino-terminal end), helix H and helix I, in addition to CBS2 of the opposing subunit ( Fig. 4 and Supplementary Fig. S1 ). Further, mutation of several residues in the region of the extracellular junction between helices F and G has profound effects on ClC-1 gating [28] , [40] , [41] , [42] . It therefore appeared likely that helix G may act as an intermediary for the coordination of common gating between the channel pore and the subunit interface. Our inactivated ClC-1 model revealed a potential bifurcated salt bridge linking residues R300 and R304 of helix I to residue D265 of helix G ( Fig. 4 ). Apart from acting as a molecular ‘scaffold’ between helix G and the subunit interface, we speculated that translation of helix G with respect to the subunit interface during common gating could alter the geometry of this network. 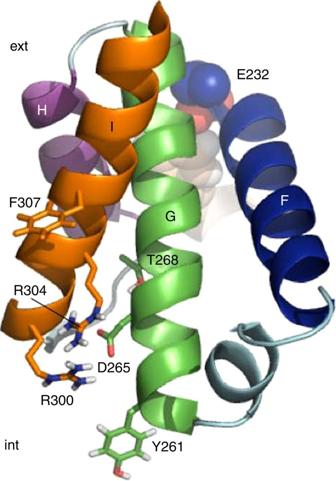Figure 4: A potential bifurcated salt bridge linking helices G-I. Inactivated ClC-1 model showing the relationship between helices F (blue), G (green), H (magenta) and I (orange); depicted in cartoon format. Extracellular (ext) and intracellular (int) faces of the membrane are indicated. Reside E232 (Eext) is shown as space-fill spheres, and residues D265, R300 and R304 are shown as sticks colored by atom type. Figure 4: A potential bifurcated salt bridge linking helices G-I. Inactivated ClC-1 model showing the relationship between helices F (blue), G (green), H (magenta) and I (orange); depicted in cartoon format. Extracellular (ext) and intracellular (int) faces of the membrane are indicated. Reside E232 (E ext ) is shown as space-fill spheres, and residues D265, R300 and R304 are shown as sticks colored by atom type. Full size image To investigate this possibility we first examined the functional consequences of charge-reversal and charge-swap mutations of the participant residues ( Table 1 and Supplementary Fig. S4 ). For the purpose of comparison we focused on the voltage dependence of gating curves, as the half-saturation values could be compared between mutants to disclose interactions between the fixed charges on the respective side chains. The basis of this analysis is that in the event that two mutations affect gating independently, the V 1/2 of double mutant gating curves should be calculable from the excursions from WT V 1/2 introduced by the single mutations. Alternatively, unpredictable V 1/2 of the double mutant would reflect interaction between the residues. Analysis of charge-reversal and charge-swap mutations showed unpredictable voltage dependence, indicating interactions between D265 and both R300 and R304; however additive effects on voltage dependence suggested no significant interaction between R300 and R304 during protopore gating ( Table 1 ). In contrast, for common gating there were significant and promiscuous interactions between all three charged residues in the network ( Table 1 ). Mutation Y261C, which is in the vicinity of these residues but is not predicted by our model to be involved in helix G–I interactions ( Fig. 4 ), has no effect on ClC-1 gating [43] . Nearby myotonic mutations F307S (helix I) and T268M (helix G) affect ClC-1 gating [24] ; however, our modelling studies suggested that the effect of these mutations is independent from the salt–bridge interaction ( Fig. 4 ). To confirm the specificity of our analysis we applied the same approach to examine inter-helical interactions between D265 and F307, and T268 and residues R300 and R304. Despite robust expression of both parental mutants, D265R/F307S mutants were non-functional, suggesting defective protein folding or trafficking. However, in keeping with our observations the voltage dependence of T268M/R300D/R304D mutant channels was predictable from the voltage dependence of the parental mutants, confirming that the residues do not interact ( Supplementary Table S2 ). Our results therefore indicate that a bifurcated salt–bridge linking helices G and I is important for gating. Table 1 A bifurcated salt bridge linking helices G-I is important for gating. Full size table We further examined these interactions by quantifying the interaction energy between charged species using a thermodynamic mutant-cycle approach [44] . The results of this analysis supported our previous experiments ( Table 2 and Supplementary Fig. S5 ). During protopore gating the interaction energy calculated for the R300 and D265 ion-pair was relatively small (approximately −1 kJ mol −1 ), and in the absence of the fixed charge on R304 there was no discernable interaction between residues R300 and D265 ( Table 2 ). Moreover, there was no interaction between R300 and R304. In contrast, common gating transitions coincided with significant, and roughly equivalent interactions between all three species (approximately −2 to 3 kJmol −1 ) and convincingly coincided with repulsion between R300 and R304 (approximately +2 kJ mol −1 ) ( Table 2 ). Table 2 Mutant-cycle analysis reveals conformational changes during common gating. Full size table NAD + inhibition of ClC-1 Y578 mutants Intracellular metabolites such as ATP and NAD + affect ClC-1 function by shifting the voltage dependence of common gating to more positive potentials and simultaneously reducing the minimum value of common gating curves [45] , [46] , [47] , [48] , [49] , [50] . These molecules bind to tandem CBS domains, which form the predominant structural feature of the extensive ClC-1 intracellular carboxy terminus. As the CBS domains are not directly exposed to the membrane voltage it is most likely that they affect gating allosterically. Mutations in CBS 2 affect ClC-1 common gating to a greater extent than mutations in CBS1 [46] , [51] . Our modelling studies suggest this is because contact between the membrane-embedded channel domain and intracellular CBS domains occurs exclusively in the region of CBS2 ( Fig. 5a and Supplementary Fig. S1 ). Helix R, which carries Y578 at its amino-terminal end, makes contact with CBS2 both directly and indirectly via extensive contacts through the region linking helix R to CBS 1 ( Fig. 5a ). It therefore appeared possible that signalling from the CBS domains could modulate common gating by affecting the conformation of Y578. Confirming this suspicion, common gating of Y578 mutant channels was largely unaffected by 3 mM intracellular NAD + ( Fig. 5b,c ). 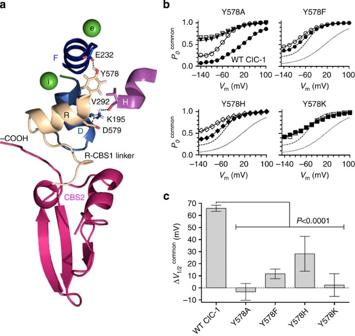Figure 5: Residue Y578 is a critical mediator of NAD+inhibition. (a) Depicts the relationship between helices D (light blue), F (blue), H (magenta), R (yellow) and CBS2 (red) in the inactivated ClC-1 model. The side chains of residues K195, E232 (Eext), V292, Y578 (Ycen) and D579, in addition to the backbone atoms of V292, are depicted as sticks coloured by atom type. Anion-binding sitesSext(e) andSint(i) are depicted as green spheres. Dashed lines represent possible polar interactions between residues. (b) Common gating curves for WT ClC-1 and Y578 mutants in the absence (open symbols) and presence (filled symbols) of 3 mM intracellular NAD+. All data are means and s.e.m. and solid lines are fits of equation (1) to the experimental data points. Dashed and dotted lines represent WT ClC-1 curves, as shown in the first figure of this panel, and are included for the purpose of comparison. (c) The mean shift of the voltage dependence of common gating curves (ΔV1/2common) by 3 mM intracellular NAD+. Data are means and linearly propagated values of s.e.m. For measurements with 3 mM NAD+n=5 (WT ClC-1), 5 (Y578A), 5 (Y578F), 3 (Y578H) and 4 (Y578K) (separate experiments). Statistical significance (P<0.0001) was determined by one-way ANOVA. Figure 5: Residue Y578 is a critical mediator of NAD + inhibition. ( a ) Depicts the relationship between helices D (light blue), F (blue), H (magenta), R (yellow) and CBS2 (red) in the inactivated ClC-1 model. The side chains of residues K195, E232 (E ext ), V292, Y578 (Y cen ) and D579, in addition to the backbone atoms of V292, are depicted as sticks coloured by atom type. Anion-binding sites S ext (e) and S int (i) are depicted as green spheres. Dashed lines represent possible polar interactions between residues. ( b ) Common gating curves for WT ClC-1 and Y578 mutants in the absence (open symbols) and presence (filled symbols) of 3 mM intracellular NAD + . All data are means and s.e.m. and solid lines are fits of equation (1) to the experimental data points. Dashed and dotted lines represent WT ClC-1 curves, as shown in the first figure of this panel, and are included for the purpose of comparison. ( c ) The mean shift of the voltage dependence of common gating curves (Δ V 1/2 common ) by 3 mM intracellular NAD + . Data are means and linearly propagated values of s.e.m. For measurements with 3 mM NAD + n =5 (WT ClC-1), 5 (Y578A), 5 (Y578F), 3 (Y578H) and 4 (Y578K) (separate experiments). Statistical significance ( P <0.0001) was determined by one-way ANOVA. Full size image A molecular pathway linking NAD + binding to Y578 Identification of residue Y578 as a critical determinant of NAD + inhibition gave us scope to investigate the pathway linking intracellular binding events to common gating. Our inactivated model suggested that, apart from the direct interaction with Y578, V292 makes contact with helix D by way of an apparent hydrogen bond between K195 and the backbone oxygen of V292 ( Fig. 5a ). Significantly, at its carboxy terminus, helix D also appears to make direct contact with CBS2 (refs 13 , 50 ). Moreover, K195 also appears to form a salt bridge with the residue neighbouring Y578, residue D579 ( Fig. 5a ). We speculated that this network could be important for relaying conformational changes commensurate with NAD + binding to residue Y578. Charge-reversal mutations underlined the importance of this linkage. Both K195D and D579K mutant channels had altered gating ( Fig. 6 and Supplementary Table S3 ). K195D mutant channels had reduced common gating ( Fig. 6b ), and were weakly sensitive to intracellular NAD + ( Fig. 6c ). In contrast, D579K mutant channels had common gating curves that were shifted to more positive voltages, and had minimum values that were lower than WT ClC-1 ( Fig. 6b ). D579K mutant channels retained sensitivity to intracellular NAD + ; however, they were less potently inhibited than WT ClC-1 ( Fig. 6b,c ). Common gating of double mutant K195D/D579K channels showed sensitivity to 3 mM NAD + that was essentially the same as the D579K mutant ( Fig. 6b,c ). In the instance that the mutations affected NAD + sensitivity independently, we would expect that double-mutant channels would be less sensitive to NAD + than either of the parental single-mutants. Supporting this hypothesis, mutation G200R on helix D also reduces sensitivity to intracellular NAD [50] , and G200R/D579K mutant channels were less sensitive to 3 mM NAD that either of the parental mutants ( Supplementary Fig. S6 ). Our results therefore indicate that the K195–D579 interaction is important for the inhibition of ClC-1 common gating by intracellular NAD + . 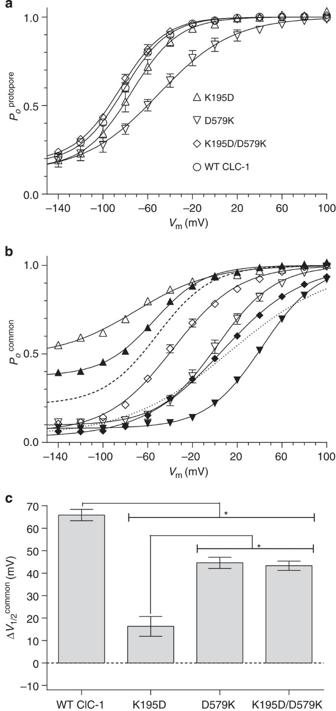Figure 6: An ion-pair interaction between K195 and D579 is important for NAD+signalling. (a) Protopore and (b) common gating curves for K195 and D579 mutant channels (open symbols). Also shown in panel (b) are common gating curves in the presence of 3 mM intracellular NAD+(filled symbols). Data are means and s.e.m., and solid lines represent fits of equation (1) to experimental data points. (c) Mean ΔV1/2commonof K195 and D579 mutant channels by 3 mM intracellular NAD+. Data are means and linearly propagated values of s.e.m. For measurements with 3 mM NAD+n=5 (WT ClC-1), 5 (K195D), 3 (D579K) and 3 (K195D/D579K) separate experiments. Asterisks denote statistical significance determined by one-way ANOVA (P<0.0001).n=3 (K195D, K195D/D579K, D579K (3NAD+), K195D/D579K (3NAD+),n=4 (WT ClC-1, D579K) orn=5 (WT (3NAD+), K195D (3NAD+)). Parameters of the fits of equation (1) to experimental data points for this figure are listed inSupplementary Table S3. Figure 6: An ion-pair interaction between K195 and D579 is important for NAD + signalling. ( a ) Protopore and ( b ) common gating curves for K195 and D579 mutant channels (open symbols). Also shown in panel ( b ) are common gating curves in the presence of 3 mM intracellular NAD + (filled symbols). Data are means and s.e.m., and solid lines represent fits of equation (1) to experimental data points. ( c ) Mean Δ V 1/2 common of K195 and D579 mutant channels by 3 mM intracellular NAD + . Data are means and linearly propagated values of s.e.m. For measurements with 3 mM NAD + n =5 (WT ClC-1), 5 (K195D), 3 (D579K) and 3 (K195D/D579K) separate experiments. Asterisks denote statistical significance determined by one-way ANOVA ( P <0.0001). n =3 (K195D, K195D/D579K, D579K (3NAD+), K195D/D579K (3NAD+), n =4 (WT ClC-1, D579K) or n =5 (WT (3NAD+), K195D (3NAD+)). Parameters of the fits of equation (1) to experimental data points for this figure are listed in Supplementary Table S3 . Full size image Our experiments strongly suggest that hydrogen bonding between the carboxylate group of E ext and the phenolic hydroxyl group of Y cen has a pivotal role in common gating of ClC channels. The importance of residue E232 for ClC-1 common gating has been established elsewhere [27] , [28] , [52] . The data presented here expound a novel role for Y578 in ClC-1 common gating. Mutation of Y cen affected common gating of ClC-1 and ClC-0 ( Fig. 2 ), predictably modulated Zn 2+ inhibition of ClC-1 common gating depending on the species replacing Y578 ( Fig. 3 ) and abrogated NAD + modulation of ClC-1 common gating ( Fig. 5 ). We therefore propose that the final effector of ClC common gating is a ‘pincer’ occlusion of S cen where the carboxylate group of E232 forms a hydrogen bond with the phenolic hydroxyl group of Y578 ( Fig. 1c and Supplementary Figs S7 and S8 ). From comparison with the mechanism proposed by Feng et al. [13] for proton transport in ClC antiporters, it is possible that protonation of E232 in this conformation leads to opening of the common gate and H + transport from the intracellular to the extracellular solution [2] , [30] . The H + transport pathway of ClC-1 is unknown, as the intracellular glutamate residue proposed to form the intracellular H + transport pathway in Cl − /H + antiporters [36] is not conserved in ClC channels ( Supplementary Fig. S1 ). Intriguingly this glutamate residue is not conserved in CmClC antiporters either, suggesting the existence of an alternate H + transport pathway [13] . Lisal and Maduke [53] have suggested that another highly conserved glutamate residue on helix H, E291 ( Supplementary Fig. S1 ), may be part of the H + transport pathway. However, our inactivated model suggests that the carboxylate groups of E232 and E291 are separated by ~14 Å ( Supplementary Fig. S7 ). An alternative H + transport mechanism that has been proposed for ClC-0 channels is direct protonation of E ext by a ‘water-wire’ pathway [54] . The current study does not address conformational changes across the subunit interface; however, a schematic overview of the rearrangements we propose to link the channel pore to the subunit interface is shown in Supplementary Fig. S8 . Our results suggest that the interaction between residues D265 and R300 arises due to ‘positioning’ of D265 via interaction with R304 during protopore gating, as there was no significant interaction in the absence of the fixed charge at position 304 and no significant interaction between residues R300 and R304 ( Table 1 ). With common gating transitions, however, interactions between all three charged species were roughly symmetrical, indicating reconfiguration of the geometry of the salt bridge ( Table 1 ). Our experiments therefore suggest translation of helix G with respect to helix I during common gating transitions. Concurrently, translation of helix G creates a binding site for Zn 2+ at the extracellular end of helix G, where Zn 2+ binding traps E232 in occupancy of S cen ( Supplementary Fig. S8 ). All mammalian ClC proteins have an acidic residue at the position corresponding to D265, and a basic residue at the position equivalent to R304 of ClC-1 ( Supplementary Fig. 1 ). Residue R300 is conserved in ClC-0, ClC-1 and ClC-2, in which a common gating mechanism has been unambiguously demonstrated [14] , [15] , [16] , [17] , [18] , [55] . Curiously, some ClC proteins that are unequivocally (ClC-4 and 5) (refs 6 , 7 ), or by way of sequence similarity (ClC-3), assumed to be anion/H + exchangers also have a basic residue at the equivalent position to R300 in ClC-1 ( Supplementary Fig. S1 ), suggesting equivalent interactions to those identified here. One possible candidate is ClC-5; however, like ClC-ec1 (refs 56 , 57 ), individual ClC-5 monomers appear to competently mediate coupled Cl − /H + transport without cooperative interactions with the opposing subunit [58] . Like ClC-1 common gating however [46] , ClC-5 function is regulated by intracellular adenosine nucleotides [59] . One possibility is that interactions linking ClC-5 helices G and I may be important for this regulatory mechanism. We have shown that residue Y578 is critical for the modulation of ClC-1 common gating by intracellular NAD + , and that the molecular pathway linking signalling from the intracellular domains to Y578 involves an ion-pair interaction between residues K195 on helix D and D579 on helix R ( Fig. 6 ). NAD + inhibition of K195D/D579K mutant channels was reduced with respect to the inhibition of WT ClC-1 ( Fig. 6c ), and although both mutations affected the voltage dependence of common gating, voltage dependence of double mutant channels reflected separate effects of the individual mutations ( Supplementary Table S3 ). One possibility that could account for these observations is disruption of the interaction between K195 and the backbone oxygen atom of V292 that was suggested by our modelling studies ( Fig. 5a ). Another possibility is that NAD + binding to the CBS domains is also relayed to the membrane-embedded channel domain by alternate pathways. Significantly, all mammalian ClC proteins, in addition to CmClC, have intracellular CBS domains and all have a basic amino acid at the position corresponding to K195 of ClC-1 and an acidic residue at the position corresponding to D579 ( Supplementary Fig. S1 ), suggesting that this signalling pathway may be conserved. Our experiments indicate that the occlusion of the central anion-binding site of the channel pore by the side chains of residues E232 and Y578 is a critical determinant of ClC-1 common gating. Our results further cement the functional convergence linking channel function and coupled anion/H + transport in the ClC protein family [11] . In accord with the model for coupled anion/H + transport proposed by Feng et al. [13] , our findings suggest that the principal difference between the seemingly disparate mechanisms of coupled transport and dissipative Cl − flux in the ClC family lie in the energy profile of the Cl − permeation pathway [13] . Homology modelling Homology models of ClC-1 were built using the published crystal structure of the homologous regions of ClC-ec1 (PDB id: 1OTS) and its E148Q mutant (PDB id: 1OTU) [8] , and CmClC (PDB id: 3ORG) [13] . In the region modelled ClC-1 and ClC-ec1 share 21% identical residues and 34% sequence similarity, and ClC-1 and CmClC share 30% identical residues and 51% sequence similarity. For ClC-ec1 based models residues K98–W595 of ClC-1, corresponding to ClC-ec1 residues R17–Q460, were modelled on ClC-ec1 coordinates. The extensive intracellular C terminus of ClC-1 was omitted from these models because ClC-ec1 does not have this domain. For the CmClC based ‘inactivated’ ClC-1 model residues V110–G872, corresponding to residues S88–N710 of CmClC, were modelled on the CmClC coordinates. ClC-1 contains a large insertion in the intracellular region of the protein linking CBS 1 and CBS 2 (R669–C820), with respect to CmClC. Critically, the region linking CBS 1 and 2 is unresolved in ClC CBS domain structures, including ClC-0 residues 619–660 (PDB id: 2D4Z) [60] , ClC-Ka residues 606–612 (PDB id: 2PFI) [61] and CmClC residues V600 – V656 (PDB id: 3ORG) [13] . Thus, the corresponding region of ClC-1, from H664–S818, was excluded from the model. Sequence alignments of the relevant protein regions were generated using TCoffee [62] and the ClC-1 models were threaded on to the appropriate structural coordinates using Swiss-Model, followed by energy minimization in SwissPDB viewer [63] . The quality of models was assessed using Verify3D [64] and found to be satisfactory. The final model was examined and figures were prepared using MacPymol 1.4.1.The CmClC and ClC-ec1-based ClC-1 models are available on request to the authors. Electrophysiology and data analysis Human ClC-1 and Torpedo marmorata ClC-0 were expressed from pCDNA3.1 expression vector in tsa201 cells (a modified HEK293 cell line) by transient transfection using Fugene 6 transfection reagent (Promega) according to the manufacturer’s specifications. For some experiments ClC-0 was expressed in HEK293 cells due to excessive whole-cell currents in tsa201 cells. Patch–clamp experiments were conducted in whole-cell configuration at room temperature (23±1 °C), 24–48 h after transfection, using an Axopatch 200B patch-clamp amplifier and Digidata 1322A A/D board controlled by AxographX ( http://www.axograph.com ) software. Currents obtained at a sampling frequency of 10 kHz were filtered at 5 kHz, and recorded using AxographX. Offline analysis was conducted using AxographX, Microsoft Excel 11.6.5 and GraphPad Prism 6.0 software. During experiments, cells were continuously superfused with bath solution containing (mM): NaCl, 140; CsCl, 4; CaCl 2 , 2; MgCl 2 , 2; HEPES, 10; adjusted to pH 7.4 with NaOH. For Zn 2+ inhibition studies, 1 mM ZnSO 4 was added to the bath solution, and during experiments rapid solution exchange was achieved using a SF-77 fast-solution exchanger (Warner instruments). The standard pipette solution contained (mM): CsCl, 40; Cs glutamate, 80; EGTA-Na, 10; HEPES, 10; adjusted to pH 6.8 with NaOH. For experiments with ClC-0, intracellular pH was adjusted to pH 7.2. Nicotinamide adenine dinucleotide (NAD + ) was purchased from Sigma-Aldrich, and a stock solution was made at a concentration of 100 mM in distilled water and stored at −20 °C. Working solutions containing NAD + were made fresh on the day of the experiment and used immediately. Patch pipettes had resistance of 1–3 MΩ when filled with the above pipette solution. Series resistance did not exceed 5 MΩ and was 85–90% compensated. After rupturing the cell membrane and achieving the whole-cell configuration, no less than 5 min was allowed for the pipette solution to equilibrate with the intracellular solution before current recordings were made. ClC-1 channel activity was assessed using the same methods as detailed elsewhere [45] , [46] , [47] . Briefly, channel open probability ( P o channel ) and open probability of the common gate ( P o common ) were determined from tail-current amplitudes, measured at −100 mV, following a 300-ms test pulse. To isolate P o common , a 400 μs pulse to +170 mV was inserted between test and tail pulses to fully activate the protopore gates [40] . The cell membrane was held at −30 mV for 4 s in between successive iterations of the voltage protocol. Open probability of the protopore gates ( P o protopore ) was calculated by dividing P o channel by P o common . For ClC-0 experiments, open probability of the protopore gates was calculated from tail current amplitudes, measured at −100 mV, following a 100 ms test pulse. Activation of the ClC-0 common gate was determined from tail current amplitudes measured at +40 mV, following a 3.5 s test pulse. The cell membrane was held at −30 mV for 10 s in between successive iterations of the voltage protocol. Gating curves ( P o ( V )) were constructed by fitting experimental data points with a modified Boltzmann distribution [17] , [40] : where P min is the minimum open probability, V is membrane voltage, V 1/2 is the half-saturation voltage and k is the slope factor. For double- and triple-charge-swap mutations measured values of V 1/2 were analysed for significant statistical difference with respect to expected values, calculated assuming independent effects of single mutations, using unpaired t tests. For experiments comparing NAD + sensitivity between mutants, statistical significance was assessed using one-way ANOVA. The time course of Zn 2+ inhibition was examined by measuring the instantaneous current amplitude following a 10 ms pulse to −100 mV, from a holding potential of −30 mV, which was applied at 4-s intervals. Zn 2+ inhibition data were normalized to the current amplitude immediately preceding the application of Zn 2+ and data were discarded if series resistance changed by >10% during the course of the experiment. To quantitatively assess the interaction energy between the charged side chains, a double or triple mutant-cycle strategy was adopted [44] . Both protopore and common gating of ClC-1 were independently examined. Gating curves, constructed using equation (1), were used to calculate Δ G 0mV , the free energy of channel gating at zero voltage, according to: where F is Faraday’s constant, V 1/2 is the half-maximal activation voltage derived from equation (1), and z is the elementary gating charge, calculated from the slope factor, k , derived from equation (1), according to: where R is the universal gas constant, T is temperature and F is Faraday’s constant. The interaction energy, ΔΔ G interact , between ion-pairs was calculated as: where Δ G 0mV (WT) is the free energy of activation of the wild-type channel, Δ G 0mV (AB) is the free energy of activation of the double mutant channel, and Δ G 0mV (A) and Δ G 0mV (B) are the free energies of activation of the respective single mutations. Linearly propagated errors were reported as s.e.m., and values of ΔΔ G interact ±s.e.m. were examined for statistical significance with respect to zero energy using a single-sample t test, with degrees of freedom= n WT + n A + n B + n AB −4, where n is the number of separate experiments for WT, single-, double- or triple-mutant channels. How to cite this article: Bennetts, B. and Parker, M.W. Molecular determinants of common gating of a ClC chloride channel. Nat. Commun. 4:2507 doi: 10.1038/ncomms3507 (2013).